Realistic control of network dynamics The control of complex networks is of paramount importance in areas as diverse as ecosystem management, emergency response and cell reprogramming. A fundamental property of networks is that perturbations to one node can affect other nodes, potentially causing the entire system to change behaviour or fail. Here we show that it is possible to exploit the same principle to control network behaviour. Our approach accounts for the nonlinear dynamics inherent to real systems, and allows bringing the system to a desired target state even when this state is not directly accessible due to constraints that limit the allowed interventions. Applications show that this framework permits reprogramming a network to a desired task, as well as rescuing networks from the brink of failure—which we illustrate through the mitigation of cascading failures in a power-grid network and the identification of potential drug targets in a signalling network of human cancer. Complex systems such as power grids, cellular networks and food webs are often modelled as networks of dynamical units. In such complex networks, a certain incidence of perturbations and the consequent impairment of the function of individual units—whether power stations, genes or species—are largely unavoidable in realistic situations. While local perturbations may only rarely disrupt a complex system, they can propagate through the network as the system accommodates to a new equilibrium. This in turn often leads to system-wide reconfigurations that can manifest themselves as genetic diseases [1] , [2] , power outages [3] , [4] , extinction cascades [5] , [6] , traffic congestions [7] , [8] and other forms of large-scale failures [9] , [10] . A fundamental characteristic of most large complex networks, both natural and man-made, is that they operate in a decentralized way. On the other hand, such networks have generally either evolved or been engineered to inhabit stable states in which they perform their functions efficiently. The existence of stable states indicates that arbitrary initial conditions converge to a relatively small number of persistent states, which are generally not unique and can change in the presence of large perturbations. Because complex networks are decentralized, upon perturbation the system can spontaneously go to a state that is less efficient than others available. For example, a damaged power-grid undergoing a large blackout may still have other stable states in which no blackout would occur, but the perturbed system may not be able to reach those states spontaneously. We suggest that many large-scale failures are determined by the convergence of the network to a ‘bad’ state rather than by the unavailability of ‘good’ states. Here we explore the hypothesis that one can design physically admissible compensatory perturbations that can be used to direct a network to a desirable state even when it would spontaneously go to an undesirable (‘bad’) state. An important precedent comes from the study of metabolic networks of single-cell organisms, where perturbations caused by genetic or epigenetic defects can lead to non-viable strains. The knockdown or knockout of specific genes has been predicted to mitigate the consequences of such defects and often recover the ability of the strains to grow [11] . Another precedent comes from the study of food-web networks, where perturbations caused by human or natural forces can lead to the subsequent extinction of multiple species. Recent research predicts that a significant fraction of these extinctions can be prevented by the targeted suppression of specific species in the system [12] . These findings have analogues in power grids, where perturbations caused by equipment malfunction/damage or operational errors can lead to large blackouts, but appropriate shedding of power can substantially reduce subsequent failures [13] , [14] . Therefore, the concept underlying our hypothesis is supported by recent research on physical [15] , [16] , biological [11] , [17] and ecological networks [12] . The question we pose is whether compensatory perturbations can be systematically identified for a general network of dynamical units. Control strategy for networks Our solution to this problem is based on the insight that associated with each desirable state there is a region of initial conditions whose trajectories converge to it—the so-called ‘basin of attraction’ of that state. Given a network that is at (or will approach) an undesirable state, the conceptual problem is thus equivalent to identifying a perturbation to the state of the system that can bring it to the attraction basin of the desired stable state (the target state). Once there, the system will evolve spontaneously to the target. However, such perturbations must be physically admissible and are, therefore, subject to constraints—in the examples above, certain genes can be downregulated but not overexpressed, the populations of certain species can only be reduced, and changes in power flow are limited by capacity and the ability to modify the physical state of the components. Under such constraints, the identification of a point within the target’s basin of attraction is a highly non-trivial task. 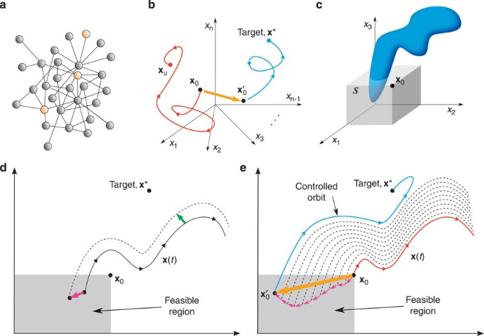Figure 1: Schematic illustration of the network control problem. (a) Network portrait. The goal is to drive the network to a desired state by perturbing nodes in acontrol set—a set consisting of one or more nodes accessible to compensatory perturbations. (b) State space portrait. In the absence of control, the network at an initial statex0evolves to an undesirable equilibriumxuin then-dimensional state space (red curve). By perturbing the initial state (orange arrow), the network reaches a new statethat evolves to the desired target statex*(blue curve). (c) Constraints. In general, there will be constraints on the types of compensatory perturbations that one can make. In this example, one can only perturb three out ofndimensions (equality constraints), which we assume to correspond to a thee-node control set, and the dynamical variable along each of these three dimensions can only be reduced (inequality constraints). This results in a set of eligible perturbations, which in this case forms a cube within the three-dimensional subspace of the control set. The network is controllable if and only if the corresponding slice of the target’s basin of attraction (blue volume) intersects this region of eligible perturbations (grey volume). (d,e) Iterative construction of compensatory perturbations. (d) A perturbation to a given initial condition (magenta arrow) results in a perturbation of its orbit (green arrow) at the point of closest approach to the target. At every step, we seek to identify a perturbation to the initial condition that brings the closest-approach point of the orbit closer to the target. (e) This process generates orbits that are increasingly closer to the target (dashed curves), and is repeated until a perturbed stateis identified that evolves to the target. The resulting compensatory perturbationx0→(orange arrow) brings the system to the attraction basin of the target without anya prioriinformation about its location, and allows directing the network to a state that is not directly accessible by any eligible perturbation. Figure 1a–c illustrates the problem that we intend to address. The dynamics of a network is best studied in the state space, where we can follow the time evolution of individual trajectories and characterize the stable states of the whole system. Figure 1a represents a network that would spontaneously go to an undesirable state, possibly due to an external perturbation, and that we would like to bring to a desired stable state by intentionally perturbing at most three of its nodes (highlighted). Figure 1b shows how this perturbation, changing the state of the system from x 0 to , would lead to an orbit that asymptotically goes to the target state. As an additional constraint, suppose that the activity of the nodes is non-negative and can only be reduced (not increased) by this perturbation. Then, in the subspace corresponding to the nodes that can be perturbed, the set of points S that can be reached by eligible perturbations forms a cubic region, as shown in Fig. 1c . The target state itself is outside this region (and, in fact, assumed to be outside the subspace of the three accessible nodes), meaning that it cannot be directly reached by any eligible perturbation. However, its basin of attraction may have points inside the region of eligible perturbations ( Fig. 1c ), in which case the target state can be reached by bringing the system to one of these points; once there, the system will spontaneously evolve towards the target state. This scenario leads to a very clear conclusion: a compensatory perturbation exists if and only if the region formed by eligible perturbations overlaps with the basin of attraction of the target. Figure 1: Schematic illustration of the network control problem. ( a ) Network portrait. The goal is to drive the network to a desired state by perturbing nodes in a control set— a set consisting of one or more nodes accessible to compensatory perturbations. ( b ) State space portrait. In the absence of control, the network at an initial state x 0 evolves to an undesirable equilibrium x u in the n -dimensional state space (red curve). By perturbing the initial state (orange arrow), the network reaches a new state that evolves to the desired target state x * (blue curve). ( c ) Constraints. In general, there will be constraints on the types of compensatory perturbations that one can make. In this example, one can only perturb three out of n dimensions (equality constraints), which we assume to correspond to a thee-node control set, and the dynamical variable along each of these three dimensions can only be reduced (inequality constraints). This results in a set of eligible perturbations, which in this case forms a cube within the three-dimensional subspace of the control set. The network is controllable if and only if the corresponding slice of the target’s basin of attraction (blue volume) intersects this region of eligible perturbations (grey volume). ( d , e ) Iterative construction of compensatory perturbations. ( d ) A perturbation to a given initial condition (magenta arrow) results in a perturbation of its orbit (green arrow) at the point of closest approach to the target. At every step, we seek to identify a perturbation to the initial condition that brings the closest-approach point of the orbit closer to the target. ( e ) This process generates orbits that are increasingly closer to the target (dashed curves), and is repeated until a perturbed state is identified that evolves to the target. The resulting compensatory perturbation x 0 → (orange arrow) brings the system to the attraction basin of the target without any a priori information about its location, and allows directing the network to a state that is not directly accessible by any eligible perturbation. Full size image However, there is no general method to identify basins of attraction (or this possible overlap) in the high-dimensional state spaces typical of complex networks (even though the desired stable states themselves are usually straightforward to identify). Despite significant advances, existing numerical techniques are computationally prohibitive and analytical methods, such as those based on Lyapunov stability theorems, offer only rather conservative estimates and are not yet sufficiently developed to be used in this context [18] , [19] , [20] . Accordingly, our approach does not assume any information about the location of the attraction basins and addresses a problem that cannot be solved by existing methods from control theory, optimization or network theory ( Supplementary Discussion ). Systematic identification of compensatory perturbations The dynamics of a complex network can often be represented by a set of coupled ordinary differential equations. We thus consider an N -node network whose n -dimensional dynamical state x is governed by We focus on models of this form because of their widespread use and availability in modelling real complex networks. However, with minor modification, the approach we develop remains effective in situations that, due to stochasticity and/or parameter uncertainty, depart from idealized deterministic models ( Supplementary Discussion , Supplementary Figs S1–S3 ). The example scenario we envision is the one in which the network has been perturbed at a time before t 0 , bringing it to a state x 0 = x ( t 0 ) in the attraction basin Ω( x u ) of an undesirable state x u . We seek to identify a judiciously chosen perturbation x 0 → to be implemented at time t 0 so that belongs to the basin of attraction Ω( x *) of a desired state x *. For simplicity, we assume that x u and x * are fixed points, although the approach we develop extends to other types of attractors. In the absence of any constraints, it is always possible to perturb x 0 such that ≡ x *. However, as discussed above, usually only constrained compensatory perturbations are allowed in real networks. These constraints encode practical considerations and often take the form of mandating no modification to certain nodes, while limiting the extent and direction of the changes in others. The latter is a consequence of the relative ease of removing versus adding resources to real systems. We thus assume that the constraints on the eligible perturbations can be represented by vector expressions of the form where the equality and inequality are interpreted to apply component-wise. We propose to construct compensatory perturbations iteratively from small perturbations, as shown in Fig. 1d . Given a dynamical system in the form (1) and an initial state x 0 at time t 0 , a small perturbation δ x 0 evolves in time according to δ x ( t )= M ( x 0 , t )· δ x 0 . The matrix M ( x 0 , t ) is the solution of the variational equation d M /d t = D F (x)· M subject to the initial condition M ( x 0 , t 0 )=1. We can use this transformation to determine the perturbation δ x 0 to the initial condition x 0 (at time t 0 ) that, among the admissible perturbations, will render x ( t c )+ δ x ( t c ) closest to x * ( Fig. 1d ), where t c is the time of closest approach to the target along the orbit. Large perturbations can then be built up by iterating the process: every time δ x 0 is calculated, the current initial state, , is updated to + δ x 0 , and a new δ x 0 is calculated starting from the new initial state ( Fig. 1e ). A visualization of this iterative procedure in two dimensions can be found in the Supplementary Information ( Supplementary Discussion , Supplementary Fig. S4 , Supplementary Movie ). Before proceeding, we stress that the compensatory perturbation—the only intervention to be actually implemented in the network—is defined by the sum of all δ x 0 . After each iteration, we test whether the new state reaches the target (Methods). If so, a compensatory perturbation has been found and is given by − x 0 . Now, it may be the case that no compensatory perturbation can be found, for example, if the feasible region S does not intersect the target basin Ω( x *). To account for this, we automatically terminate our search if the system is not controlled within a sufficiently large number of iterations (Methods). We have, however, benchmarked our approach using randomly generated networks in which compensatory perturbations are known to exist under the given constraints ( Supplementary Discussion ). Our method succeeds in identifying them in 100% of cases, thus providing confidence that the approach introduced here can indeed be used to control a network when it is theoretically possible to do so. We note that our approach is effective even when it has to cross multiple attraction basins ( Supplementary Fig. S4b ) and when the basin boundaries are complex ( Supplementary Discussion , Supplementary Figs S5 and S6 ). The above benchmark also confirms the efficiency of our algorithm ( Supplementary Figs S7 and S8 ), for which the theoretical running time is O ( n 2.5 ), where n is the number of dynamical variables in the network ( Supplementary Discussion ). Computationally, this is not onerous, especially since the control of a network requires the identification of only one compensatory perturbation. This should be contrasted with the time that would be required to determine the basin of attraction at fixed resolution by direct sampling of the state space. Application to the identification of therapeutic interventions We apply our approach to the identification of potential therapeutic targets in a form of human blood cancer (large granular lymphocytic leukaemia) caused by the abnormal survival of certain white blood cells (cytotoxic T cells). These T cells are part of the immune system and are produced to attack infected or dysfunctional cells. Under normal conditions, once the compromised cells have been removed, a significant portion of the T cells undergo programmed cell death (apoptosis). The disease, T-LGL leukaemia, results precisely from the failure of T cells to undergo apoptosis, and the consequent negative impact they have on normal cells of the body [21] . The identification of potential therapeutic interventions is important as, at present, there is no curative treatment for this disease. To formulate the problem, we use the 60-node survival signalling network model of T cells reconstructed and validated in Zhang et al. [22] , where nodes correspond to proteins, transcripts, inputs (for example, external stimuli), and cellular concepts (for example, apoptosis). The state of each node is represented by a continuous variable between 0 and 1 (Methods). According to this model, normal and cancer states correspond to two different types of stable steady states. Potential curative interventions are those that can bring the system from a cancerous or precancerous state (those in the attraction basin of a cancer state) to the attraction basin of the normal state, which leads to apoptosis. Previous experimental and computational studies have identified 19 nodes in this network as promising targets for curative interventions based on single, permanent reversals of the corresponding (binary) gene or protein activity in the cancer state [23] . The question we pose is whether novel interventions exist among the remaining nodes in the network (potentially involving multiple nodes), and furthermore, whether they can be effective with only the temporary , one-time perturbations considered here. 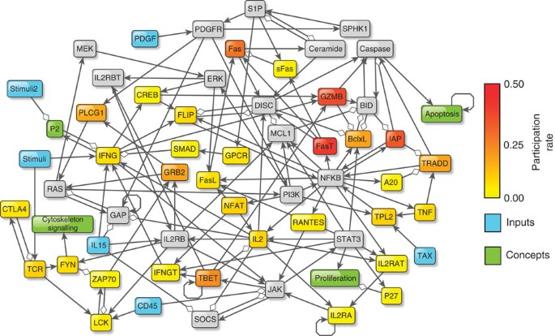Figure 2: T-cell survival signalling network governing the development of T-LGL leukemia. Conceptual nodes, input nodes and previously identified potential therapeutic targets are shown in green, blue and grey, respectively. The edges represent interactions, with the arrowheads and diamonds corresponding to activation and inhibition, respectively. The inhibitory edges that exist between Apoptosis and all non-input nodes are not shown for clarity. The 31 nodes coloured yellow–red represent proteins and transcripts considered in our search for novel therapeutic targets, and are colour-coded based on the frequency with which they appear (participation rate) in the smallest control sets that we identify to successfully direct the network from a precancerous state to the attraction basin of the normal cell state. Given a compensatory perturbationx0→(such thatx0is a precancerous state andlies in the basin of attraction of the normal cell state), we find small control sets by first sorting the 31 nodes under consideration in decreasing order based on the amount they were perturbed, and then searching for a new compensatory perturbation involving only the firstknodes in this list. Through bisection on the numberk, we are able to quickly converge to the ‘minimal’ control set (with respect to this ordering) that can be used to rescue the given precancerous state. This procedure is remarkably effective at producing small control sets—the average size is 3.4 (with s.d. 3.7). Figure 2 shows the 19 previously characterized targets (grey), 10 nodes representing static inputs (blue) or concepts (green), and the remaining 31 nodes (yellow–red) that we use to search for novel interventions. Figure 2: T-cell survival signalling network governing the development of T-LGL leukemia. Conceptual nodes, input nodes and previously identified potential therapeutic targets are shown in green, blue and grey, respectively. The edges represent interactions, with the arrowheads and diamonds corresponding to activation and inhibition, respectively. The inhibitory edges that exist between Apoptosis and all non-input nodes are not shown for clarity. The 31 nodes coloured yellow–red represent proteins and transcripts considered in our search for novel therapeutic targets, and are colour-coded based on the frequency with which they appear (participation rate) in the smallest control sets that we identify to successfully direct the network from a precancerous state to the attraction basin of the normal cell state. Given a compensatory perturbation x 0 → (such that x 0 is a precancerous state and lies in the basin of attraction of the normal cell state), we find small control sets by first sorting the 31 nodes under consideration in decreasing order based on the amount they were perturbed, and then searching for a new compensatory perturbation involving only the first k nodes in this list. Through bisection on the number k , we are able to quickly converge to the ‘minimal’ control set (with respect to this ordering) that can be used to rescue the given precancerous state. This procedure is remarkably effective at producing small control sets—the average size is 3.4 (with s.d. 3.7). Full size image We first allowed all of these 31 accessible nodes to be perturbed, under the constraints that their state variables are kept within 0 and 1, and that the other nodes are not perturbed. Because it is important to consider intermediary cell states that lead to the cancer state, we sought to identify compensatory perturbations for 10,000 such states selected from a uniform sampling of the state space. Of these, 67% are successfully rescued using our approach. As shown in Fig. 3 , a number of striking patterns emerge in the interventions we found. Most nodes are consistently suppressed, which may in part be attributed to the fact that all nodes other than Apoptosis are inactive in the target state, but this is also true for nodes that are inactive in the cancer state. In addition, there are several nodes whose activity is consistently enhanced, despite the fact that they are active in the cancer state. These counterintuitive interventions are unlikely to be identified by simple inspection of the network or its stable states. 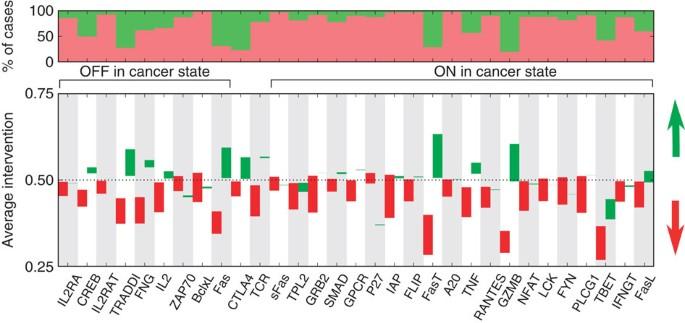Figure 3: Size and orientation of compensatory perturbations in the T-cell survival signalling network. Each column corresponds to one of the 31 nodes under consideration as potential therapeutic targets, which are ordered according to their predicted activity in the cancer state. The data represent a sample of 10,000 precancerous network states, 6,731 of which are successfully rescued through compensatory perturbations identified by our approach. The top panel shows the relative fraction of the successful interventions in which the activity of each individual node is increased (green) versus decreased (red). The corresponding colours in the bottom panel represent the average preperturbation activity and the orientation and size of the compensatory perturbation. Nodes are marked as either OFF or ON in the cancer state when their activity is ≈ 0 or ≈ 1 in that state, respectively (the only exceptions are the nodes CTLA4 and TCR, whose activity is ≈ 0.5 in the cancer state). Remarkably, the interventions are such that a number of nodes are consistently perturbed toward, rather than away from, their activity levels in the undesirable (cancer) state. Figure 3: Size and orientation of compensatory perturbations in the T-cell survival signalling network. Each column corresponds to one of the 31 nodes under consideration as potential therapeutic targets, which are ordered according to their predicted activity in the cancer state. The data represent a sample of 10,000 precancerous network states, 6,731 of which are successfully rescued through compensatory perturbations identified by our approach. The top panel shows the relative fraction of the successful interventions in which the activity of each individual node is increased (green) versus decreased (red). The corresponding colours in the bottom panel represent the average preperturbation activity and the orientation and size of the compensatory perturbation. Nodes are marked as either OFF or ON in the cancer state when their activity is ≈ 0 or ≈ 1 in that state, respectively (the only exceptions are the nodes CTLA4 and TCR, whose activity is ≈ 0.5 in the cancer state). Remarkably, the interventions are such that a number of nodes are consistently perturbed toward, rather than away from, their activity levels in the undesirable (cancer) state. Full size image We can reduce the number of nodes that are perturbed by taking advantage of the reasonable expectation that the nodes that have been perturbed by the largest amount should dominate the membership of the smallest successful control sets ( Fig. 2 ). Specifically, we find that we can rescue the same precancerous states above with an average (standard deviation) of only 3.4 (3.7) nodes. These interventions involve a small number of genes but at the same time are multi-target, which is desirable given that the cure for currently incurable diseases is believed to reside in the coordinated modulation of multiple cellular components [24] . Such interventions are prohibitively difficult to identify experimentally by exhaustive search in the absence of computational predictions such as ours. Moreover, there is a high degree of overlap between these reduced control sets ( Fig. 2 ), with nodes GZMB and FasT participating in nearly half of them. These nodes, and other frequently occurring nodes such as IAP and Fas, are attractive candidates for experimental verification. Some of these genes work in tandem, with control sets formed by FasT and Fas alone predicted to rescue over 13% of all cases. Our analysis suggests that interventions can be effective even if they are temporary , which, because they can be more easily implemented pharmacologically, are preferable to potential therapies based on permanent changes to a node state. Reprogramming in associative memory networks In an associative memory network, each memorized pattern is encoded as an attractor. An important problem in this context concerns the identification of constrained perturbations that cause the network to transition from a given pattern to a different specific pattern. To illustrate this problem, we consider a model of associative memory consisting of N identical coupled oscillators [25] , where θ i is the phase variable of oscillator i , C ij are the elements of the interaction matrix, and is the strength of the second-order coupling term. Up to translation of all oscillators by a constant phase, system (3) has 2 N fixed points, corresponding to the phase-locked solutions in which | θ j − θ i |=0 or | θ j − θ i |= π for every i and j . The attractors in this system consist of all such fixed points that are stable [25] . This way, each asymptotic state of the network is identified uniquely with a binary pattern. In order to preferentially stabilize the desired states, the network is wired according to Hebb's learning rule , where with ( i =1,..., N , μ =1,..., p ) is the set of p binary input patterns of length N to be stored [26] . As an example, we consider a network of size N =64, for ε =0.8, storing p =7 patterns that represent the letters of the word ‘NETWORK’. The resulting network is depicted in Fig. 4a . 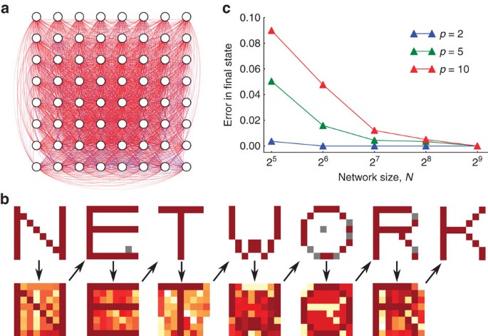Figure 4: Control in an associative memory network. (a) Wiring diagram of a network ofN=64 oscillators storing patterns representing the seven letters in the word ‘NETWORK’, where red (blue) lines denote connections of positive (negative) weight. (b) Examples of transitions between memorized patterns induced by compensatory perturbations. Taking an initial statecorresponding to a letter in the word ‘NETWORK’, we attempt to find a perturbation(downward arrows) that then causes the network to spontaneously transition to the next letter under time evolution (diagonal arrows). Each oscillator is colour-coded based on its angular distance from oscillator 1 (a,upper left), while the errors between the final state that is actually reached and the state that was targeted are indicated in grey. In each of the six cases, the control procedure successfully brings the system to the target or to a visually similar stable state with few such errors. (c) Similar analysis shows that these errors become negligible as the size of the network is increased relative to the number of stored patterns. The curves indicate the average error (measured as the fraction of mismatched pixels) between the target state and the final stable state actually reached using our control procedure. This average error is shown as a function of the network sizeN, for networks storing 2 (blue), 5 (green) and 10 (red) random patterns, with each of theNpixels having equal probability of being ±1. The coupling strength ε is 0.2, 0.4 and 0.8, respectively. Every point represents a set of 1,000 independent network realizations, each sampled once, where the initial and target states are taken at random among the stored patterns. Figure 4: Control in an associative memory network. ( a ) Wiring diagram of a network of N =64 oscillators storing patterns representing the seven letters in the word ‘NETWORK’, where red (blue) lines denote connections of positive (negative) weight. ( b ) Examples of transitions between memorized patterns induced by compensatory perturbations. Taking an initial state corresponding to a letter in the word ‘NETWORK’, we attempt to find a perturbation (downward arrows) that then causes the network to spontaneously transition to the next letter under time evolution (diagonal arrows). Each oscillator is colour-coded based on its angular distance from oscillator 1 ( a, upper left), while the errors between the final state that is actually reached and the state that was targeted are indicated in grey. In each of the six cases, the control procedure successfully brings the system to the target or to a visually similar stable state with few such errors. ( c ) Similar analysis shows that these errors become negligible as the size of the network is increased relative to the number of stored patterns. The curves indicate the average error (measured as the fraction of mismatched pixels) between the target state and the final stable state actually reached using our control procedure. This average error is shown as a function of the network size N , for networks storing 2 (blue), 5 (green) and 10 (red) random patterns, with each of the N pixels having equal probability of being ±1. The coupling strength ε is 0.2, 0.4 and 0.8, respectively. Every point represents a set of 1,000 independent network realizations, each sampled once, where the initial and target states are taken at random among the stored patterns. Full size image We seek to identify perturbations that induce transitions between the memorized patterns while only changing oscillators representing ‘off’ pixels, thereby requiring the existing pattern to be preserved. Figure 4b shows the results for initial/target state pairs corresponding to consecutive letters of ‘NETWORK’. In every case, the constraints on the eligible perturbations forbid reaching the target state directly. Nonetheless, in every case, the control procedure succeeds in identifying a perturbed initial state (bottom row) that spontaneously evolves to the target or to a similar pattern with a small number of binary errors (grey)—and which is expected to become smaller in larger networks ( Fig. 4c ). Thus, even if the basin of attraction of the target state cannot be reached by any eligible perturbation, it may nonetheless be possible to drive the network to a similar state using our control procedure. Control of desynchronization instabilities in power-grid networks In the design and operation of power-grid networks, an important consideration is the ability of the power generators to maintain synchrony following perturbations [27] , [28] . Desynchronization instabilities have in fact been implicated in cascading failures underlying major recent blackouts [29] . The state of the system is assumed to be determined by the swing equation, where N is the number of generators in the network and δ i and ω i are the phase and angular frequency of generator i , respectively. The constant H i is the inertia parameter of the generator, is the mechanical input power from the generator, and is the power demanded of the generator by the network [30] . The network structure and impedance parameters are incorporated into the matrices D ′=( ) and D ′′=( ), and the damping is accounted for by the coefficient D i . In equilibrium, and all generators operate in a synchronous state, characterized by ω 1 = ω 2 =…= ω N . We illustrate our control procedure on the New England power-grid model [31] , which operates at the nominal synchronization frequency ω s =2 π × 60 rads −1 and consists of 10 generator nodes, 39 load nodes, and 46 transmission lines ( Fig. 5a ). We implement this simple model for the parameter values given in Susuki et al. [30] . 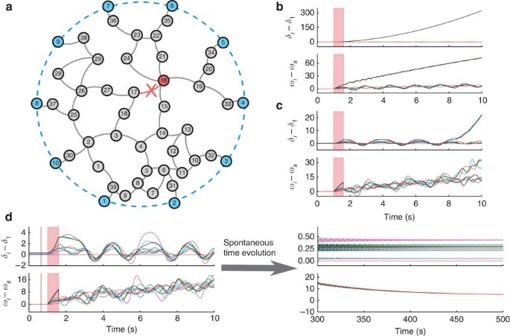Figure 5: Control of the New England power-grid test system following a fault. (a) Schematic diagram of the network. The generators (theN=10 dynamical nodes in the network) are highlighted in blue, and the non-generator nodes appear in grey. The simulated fault is on the line connecting nodes 16 and 17 (red). It consists of short-circuiting the end 16 of the line with the ground for the period 1.0–1.6 s and subsequently removing the affected line from the network. (b–d) Dynamics of the generators, characterized by the phasesδi(upper panels) and angular frequenciesωi(lower panels): (b) without any control perturbation, (c) with a naive intervention based on resetting the generators' frequencies to the frequency of the target state, and (d) with a compensatory perturbation identified by our control procedure. The fault induces a desynchronization (b), which is not remediated by the naive intervention (c), but the iterative control procedure identifies a configuration of generator frequencies that maintains bounded swings in the short term (d, left), and ultimately causes the system to evolve to the new synchronous (target) state (d, right). This simplified example was chosen to have very large frequency deviations and transient period to facilitate visualization. In a realistic setting, the interventions can be implemented by tuning the damping of the generators. Figure 5: Control of the New England power-grid test system following a fault. ( a ) Schematic diagram of the network. The generators (the N =10 dynamical nodes in the network) are highlighted in blue, and the non-generator nodes appear in grey. The simulated fault is on the line connecting nodes 16 and 17 (red). It consists of short-circuiting the end 16 of the line with the ground for the period 1.0–1.6 s and subsequently removing the affected line from the network. ( b – d ) Dynamics of the generators, characterized by the phases δ i (upper panels) and angular frequencies ω i (lower panels): ( b ) without any control perturbation, ( c ) with a naive intervention based on resetting the generators' frequencies to the frequency of the target state, and ( d ) with a compensatory perturbation identified by our control procedure. The fault induces a desynchronization ( b ), which is not remediated by the naive intervention ( c ), but the iterative control procedure identifies a configuration of generator frequencies that maintains bounded swings in the short term ( d , left), and ultimately causes the system to evolve to the new synchronous (target) state ( d , right). This simplified example was chosen to have very large frequency deviations and transient period to facilitate visualization. In a realistic setting, the interventions can be implemented by tuning the damping of the generators. Full size image For an initially steady-state solution determined by power flow calculations, we simulate single-line faults caused by short circuits to the ground for a period of 0.6 s, during which the corresponding impedance is assumed to be very small ( z =10 −9 j) and at the end of which the fault is cleared by disconnecting the line. Figure 5 shows one such fault on the line connecting nodes 16 and 17 ( Fig. 5a ) and the corresponding time evolution of the δ i and ω i for all generators in the network ( Fig. 5b–d ). By the time the fault is cleared, the generators have lost synchrony, and in the absence of any intervention, they continue accelerating away from one another ( Fig. 5b ). Nonetheless, the perturbed network admits a stable steady-state synchronous solution characterized by a new set of generator phases and a synchronization frequency only slightly different from ω s . In asking whether loss of synchrony can be averted by an appropriate compensatory perturbation following the fault, for illustrative purposes we assume that direct modification of the generator phases δ i is prohibited and only perturbations to the generator frequencies ω i are allowed. A naive approach would be to reset the generator frequencies to the corresponding values at the target state after the fault, but, for not accounting for the full 2 N dimensions of the state space, this approach fails and the system still loses synchrony, albeit at a later time ( Fig. 5c ). Using our iterative network control procedure, however, one can identify a post-fault intervention that maintains bounded generator oscillations in the short term ( Fig. 5d , left), and eventually causes the perturbed network to evolve to the desired target state ( Fig. 5d , right). Out of the 92 possible single-line fault perturbations of the type described above, 43 cause the perturbed network to evolve to an undesirable final state in which the generators have lost synchrony. Of these, 27 cases can be controlled under the constraints described above. In each of the cases in which our method fails to find a compensatory perturbation, naive heuristic interventions—specifically, resetting the generators identically to either the nominal frequency or the synchronization frequency at the target state—also fail, suggesting that these perturbed networks may be impossible to control under the given constraints. The dynamics of large natural and man-made networks are usually highly nonlinear, making them complex not only with respect to their structure but also with respect to their dynamics. Nonlinearity has been the main obstacle to the control of such systems, and this is well reflected in the state of the art in the field [32] , [33] . Progress has been made in the development of algorithms for decentralized communication and coordination [34] , in the manipulation of Boolean networks [35] , in network queue control problems [36] , and in other complementary areas. Methods have been developed for the control of networks hypothetically governed by linear dynamics [37] . However, although linear dynamics may approximate an orbit locally, control trajectories are inherently nonlocal [38] ; moreover, linear dynamics does not permit the existence of the different stable states observed in real networks and does not account for basins of attraction and other global properties of the state space. These global properties are crucial because they underlie network failures and, as shown here, provide a mechanism for network control. This can be achieved under rather general conditions by systematically designing compensatory perturbations that take advantage of the full basin of attraction of the desired state, thus capitalizing on (rather than being obstructed by) the nonlinear nature of the dynamics. Applications show that our approach is effective even when compensatory perturbations are limited to a small subset of all nodes in the network, and when constraints forbid bringing the network directly to the target state. From a network perspective, this frequently leads to counterintuitive situations in which the compensatory perturbations are in an opposite direction from that towards the target state—for example, suppressing nodes that are already less active than at the target. These results are surprising in light of the usual interpretation that nodes represent ‘resources’ of the network, to which we then intentionally (albeit temporarily) inflict damage with a compensatory perturbation. The same holds true for the converse, as demonstrated in the T-cell survival signalling network. There the goal is to induce cell death, which, counterintuitively, is often achieved through perturbation towards the (active) cancer state. From the state space perspective, the reason for the existence of such locally deleterious (beneficial) perturbations that have globally beneficial (deleterious) effects is that the basin of attraction, being nonlocal, can extend to the region of feasible perturbations even when the target itself does not. We have motivated our problem assuming that the network is away from its desired equilibrium due to an external perturbation. In particular, as shown in our example of desynchronization failures in a power-grid, our approach can be used for the real-time rescue of a network, bringing it to a desirable state before it reaches a state that can be temporarily or permanently irreversible. We suggest that this can be important for the conservation of ecological systems and for the creation of self-healing infrastructure systems. On the other hand, as illustrated in our associative memory example, our approach also applies to move the network from one stable state to another, thus providing a mechanism for ‘network reprogramming’. As a broader context to interpret the significance of this application, consider the reprogramming of differentiated (somatic) cells from a given tissue into a pluripotent stem cell state, which can then differentiate into cells of a different type of tissue. The seminal experiments demonstrating this possibility involved continuous overexpression of specific genes [39] , which is conceivable even under the hypothesis that cell differentiation is governed by the loss of stability of the stem cell state [40] . However, the recent demonstration that the same can be achieved by the temporary expression of few proteins [41] or transient administration of messenger RNA [42] indicates that the stem cell state may have remained stable (or metastable) after differentiation, allowing interpretation of the reprogramming process in the context of the interventions considered here. While induced pluripotency is an example par excellence of network reprogramming, the same concept extends far beyond this particular system. Taken together, our results provide a new foundation for the control and rescue of network dynamics and, as such, are expected to have implications for the development of smart traffic and power-grid networks, of ecosystems and Internet management strategies, and of new interventions to control the fate of living cells. Identification of compensatory perturbations We identify compensatory perturbations iteratively as follows. Given the current initial state of the network, , we integrate the system dynamics over a time window t 0 ≤ t ≤ t 0 + T to identify the time of the orbit’s closest approach to the target, t c ≡ arg min| x *− x ( t )|. We then integrate the variational equation up to this time to obtain the corresponding variational matrix, M ( t c ), which maps a small change δ x 0 to the initial state of the network to a change δ x ( t c ) in the resulting perturbed orbit at t c according to δ x ( t c )= M ( t c )· δ x 0 . This mapping is used to select an incremental perturbation δ x 0 to the current initial state that minimizes the distance between the perturbed orbit and the target at time t c , subject to the constraints (2) on the eligible perturbations, as well as additional constraints on δ x 0 to ensure the validity of the variational approximation ( Constraints on incremental perturbations , below). This selection is performed via a nonlinear optimization ( Nonlinear optimization , below). The initial condition is then updated according to → + δ x 0 , and we test whether the new initial state lies in the target's basin of attraction by integrating the system dynamics over a long time τ . If the system’s orbit reaches a small ball of radius κ around x * within this time, we declare success and recognize x 0 − as a compensatory perturbation (for the updated x ′ 0 ). If not, we calculate the time of closest approach of the new orbit and repeat the procedure, up to a maximum number I of iterations. Constraints on incremental perturbations The incremental perturbation at the point of closest approach, δ x ( t c ), selected under constraints (2) alone will generally have a non-zero component along a stable subspace of the orbit x ( t ), which will result in δ x 0 larger than δ x ( t c ) by a factor of up to , where is the finite-time Lyapunov exponent of the eigendirection corresponding to the eigenvalue of M ( x 0 , t c ) with smallest-magnitude real part. In a naive implementation of this algorithm, to keep δ x 0 small for the linear transformation to be valid, the size of δ x ( t c ) would be negligible, leading to negligible progress. This problem is avoided by optimizing the choice of δ x ( t c ) under the constraint that the size of δ x 0 is bounded above. Another potential problem is when the perturbation causes the orbit to cross an intermediate basin boundary before reaching the final basin of attraction. All such events can be detected by monitoring the difference between the linear approximation and the full numerical integration of the orbit, without requiring any prior information about the basin boundaries. Boundary crossing is actually not a problem because the closest approach point is reset at each iteration and, in particular, on the new side of the basin boundary. To assure that the method will make satisfactory progress at each iteration, we solve the optimization problem under the constraint that the size of δ x 0 is also bounded below, which means that we accept increments δ x 0 that may temporarily increase the distance from the target. These upper and lower bounds can be expressed as This can lead to due to components along the unstable subspace, but in such cases the vectors can be rescaled after the optimization. At each iteration, the problem of identifying a perturbation δ x 0 that incrementally moves the orbit toward the target under constraints (2) and (5) is then solved as a constrained optimization problem. To avoid back-and-forth oscillations, we require the inner product between the two consecutive increments δ x 0 to be positive. The resulting iterative procedure behaves well as long as , which can be assured by properly choosing ε 0 and ε 1 , where is the actual change in the orbit at t c measured when the orbit is integrated anew at the subsequent iteration. In practice, the approach does not depend critically on very accurate forecasting of δ x ( t c ) at any single iteration so long as it moves the orbit closer to the target, and it is observed to be effective for a rather wide range of parameters ε 0 and ε 1 . Nonlinear optimization The optimization step of the iterative control procedure consists of finding the small perturbation δ x 0 that minimizes the remaining distance between the target, x *, and the system orbit x ( t ) at its time of closest approach, t c . Constraints are used to define the admissible perturbations (2) and also, as described in the previous paragraph, to limit the magnitude of δ x 0 (5). The optimization problem to identify δ x 0 can then be succinctly written as: where (10) is enforced starting from the second iteration, and denotes the incremental perturbation from the previous iteration. Formally, this is a nonlinear programming problem, the solution of which is complicated by the non-convexity of the constraint (9) (and possibly (7) and (8)). Nonetheless, a number of algorithms have been developed for the efficient solution of nonlinear programming problems, among them sequential quadratic programming [43] . This algorithm solves (6) subject to (7)–(10) as the limit of a sequence of quadratic programming subproblems, in which the constraints are linearized in each substep. For all calculations, we use the sequential quadratic programming algorithm [44] implemented in the SciPy scientific programming package ( http://www.scipy.org/ ). In all systems, we use dimensionless distances. In the case of the power-grid network, this is implemented by normalizing frequency by the target frequency, which further avoids disparate scales between the frequency and phase variables. More generally, while the norm in (6) may denote the usual Euclidean norm for most systems, there is nothing in our formulation of the control procedure that prohibits optimizing closeness according to a different metric in a particular network, especially if the dynamical variables represent different quantities or are otherwise not of the same order. Values of parameters For the values of the parameters κ , τ, I , ε 0 , ε 1 and T used in the example applications of this paper, as well as criteria for choosing their values in the general case, we refer the reader to the Supplementary Methods and Supplementary Table S1 . T-cell survival signalling network The network consists of 60 nodes, 54 of which are equipped with dynamics and represent the state of the network, while 6 are static input nodes (Stimuli, TAX, CD45, PDGF, Stimuli2 and IL15) [22] , [23] . Following Zhang et al. [22] and Saadatpour et al. [23] , we set Stimuli, IL15 and PDGF at ON (one) and set TAX, CD45 and Stimuli2 at OFF (zero) for all simulations. We translate the Boolean network dynamics given in Saadatpour et al. [23] into an equivalent continuous form using the method described in Wittmann et al. [45] The state variable x i representing the activity of each node is thus allowed to assume values in the range [0,1]. The associated dynamics follows Here B i is a continuous analogue of the discrete Boolean update rule for node i , which would take the current state (ON or OFF) of all nodes as an input and output the state of node i at the next time step. The function B i is obtained via multilinear interpolation of the associated logical function between the ‘corners’ of the N -dimensional unit cube (in which the value of each node is either 0 or 1). To capture the switch-like behaviour observed in signalling circuits, the state of each node is passed through a sigmoidal (Hill-type) function f ( x )= x 4 /( x 4 + k 4 ) before it is used as an input to the continuous logical gates B i . Nodes are considered to be ON (OFF) if the associated x i is significantly above (below) the threshold k , which we take to be 0.5. The generation of the continuous model dynamics was done automatically with the software package Odefy [46] . We observe three stable fixed points in the network. One fixed point corresponds to the normal cell state (the target state in our simulations), in which the node representing apoptosis is ON and all other dynamical nodes are OFF. The two other fixed points are biologically equivalent (differing only by node P2, which can be either ON or OFF) and correspond to the cancer state. The three attractors, as defined by the associated ON/OFF states of the individual nodes, are identical to those found in Saadatpour et al. [23] . How to cite this article: Cornelius, S. P. et al. Realistic control of network dynamics. Nat. Commun. 4:1942 doi: 10.1038/ncomms2939 (2013).